Repurposing Blu-ray movie discs as quasi-random nanoimprinting templates for photon management Quasi-random nanostructures have attracted significant interests for photon management purposes. To optimize such patterns, typically very expensive fabrication processes are needed to create the pre-designed, subwavelength nanostructures. While quasi-random photonic nanostructures are abundant in nature (for example, in structural coloration), interestingly, they also exist in Blu-ray movie discs, an already mass-produced consumer product. Here we uncover that Blu-ray disc patterns are surprisingly well suited for light-trapping applications. While the algorithms in the Blu-ray industrial standard were developed with the intention of optimizing data compression and error tolerance, they have also created quasi-random arrangement of islands and pits on the final media discs that are nearly optimized for photon management over the solar spectrum, regardless of the information stored on the discs. As a proof-of-concept, imprinting polymer solar cells with the Blu-ray patterns indeed increases their efficiencies. Simulation suggests that Blu-ray patterns could be broadly applied for solar cells made of other materials. Quasi-random nanostructures [1] , [2] , [3] , [4] are abundant in nature for light manipulation purposes, such as in structural coloration in birds and insects [5] , [6] , [7] . These disordered structures have received renewed interest for photon management in a variety of engineering applications, such as highly efficient photon extraction in light-emitting diodes [8] , biomimetic structural coloration [5] , [9] and random lasing [10] , [11] . Unlike perfectly periodic [12] , [13] , [14] , [15] , [16] or totally random structures, quasi-random nanostructures can offer both broadband absorption enhancement and customizable spectral response for different photoactive materials [4] , [17] , [18] , [19] . However, very expensive fabrication processes are typically needed to create these disordered, subwavelength patterns suitable for light trapping in photonic devices. Interestingly, such patterns already exist in a mass-produced consumer product. Here we report repurposing of Blu-ray movie discs as quasi-random nanoimprinting templates. Regardless of the media’s content, the audio and video compression algorithms convert the data to a high-entropy binary sequence. After error-correcting and modulation coding, a quasi-random pattern of pits is eventually generated on the disc, which we found to be surprisingly well suited for photon management over the entire solar spectrum. As a proof-of-concept, we successfully imprinted the Blu-ray pattern onto the active layer—and subsequently to the metal electrode—of polymer solar cells, leading to higher absorption and power conversion efficiencies. In addition, we numerically demonstrate the promise of this technique for enhancing light trapping for other photoactive materials. This new insight opens up promising areas for repurposing a low-cost consumer product for a high-end, value-added application. Assessing the Blu-ray pattern for light trapping The arrangement of nanostructures within a light-trapping layer dramatically affects how photon energy is coupled into the plasmonic and waveguide modes confined in the active layer of a solar cell [20] . 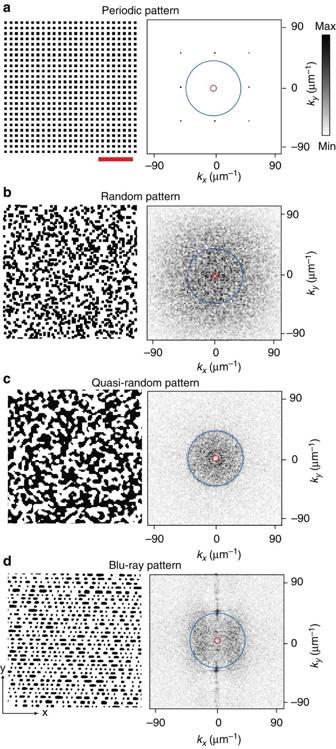Figure 1: Fourier transforms of subwavelength features arranged in periodic, random, quasi-random and Blu-ray patterns. Real space (red scale bar, 2.5 μm) and Fourier space. The circles denote the largest (blue) and smallestk-values needed to couple the entire solar spectrum (315 nm to 2.5 μm) to surface plasmons at the interface between an example photoactive layer, PTB7:PC71BM and silver electrode. (a) A periodic and (b) a random pattern yield wavevectors that are either too discretized or too diffuse to lie between the two circles, in contrast to (c) an optimized quasi-random pattern. (d) A Blu-ray pattern, obtained by thresholding an AFM image of the recording layer of a movie disc (seeSupplementary Fig. 1), produces surprisingly close-to-optimized distribution ofk-values. Figure 1 shows the Fourier transforms of subwavelength features arranged in periodic, random, quasi-random and Blu-ray patterns. The red and blue circles in Fourier space mark the k -values required to couple incoming light into the waveguide modes at the red and blue ends of the solar spectrum, respectively. Periodic ( Fig. 1a ) and random ( Fig. 1b ) patterns yield wavevectors that are either too discretized or too diffuse, respectively. On the other hand, quasi-random patterns ( Fig. 1c ) can be optimized to yield Fourier spectra that are efficient in light trapping, but these patterns are typically prohibitively expensive to manufacture. In comparison, although still containing a periodic component, the pattern on a pre-written Blu-ray movie disc ( Fig. 1d ) produces a close-to-optimized distribution of k -values. Figure 1: Fourier transforms of subwavelength features arranged in periodic, random, quasi-random and Blu-ray patterns. Real space (red scale bar, 2.5 μm) and Fourier space. The circles denote the largest (blue) and smallest k -values needed to couple the entire solar spectrum (315 nm to 2.5 μm) to surface plasmons at the interface between an example photoactive layer, PTB7:PC 71 BM and silver electrode. ( a ) A periodic and ( b ) a random pattern yield wavevectors that are either too discretized or too diffuse to lie between the two circles, in contrast to ( c ) an optimized quasi-random pattern. ( d ) A Blu-ray pattern, obtained by thresholding an AFM image of the recording layer of a movie disc (see Supplementary Fig. 1 ), produces surprisingly close-to-optimized distribution of k -values. Full size image The Blu-ray disc (BD) standard [21] was developed for high-density optical data storage, and has proven popular for distributing high-definition movies. The BD standard specifies that the track pitch and width are 320 and 130 nm, respectively, and a single bit would be 75 nm long. When recorded to a disc, the video signals are first compressed to a binary sequence with high entropy per bit (for example, according to the MPEG-4 format), whose local statistics is are very similar to those of a sequence of random, independent, unbiased coin tosses [22] . When reading data from the disc, however, very short runs of successive zeros or ones yield low signal amplitudes and very long runs are difficult to distinguish from noise due to scratches or fingerprints [21] . Therefore, an error-control modulation code is applied to the data so that the number of successive zeros or ones is between 2 and 7. When written to the disc, eventually a quasi-random pattern of islands and pits with lengths between 150 and 525 nm are generated (see a representative atomic force microscopy (AFM) image in Supplementary Fig. 1a ), whose Fourier components are surprisingly well-suited for photon management over the broad visible and near-infrared portion of the spectrum, regardless of the movie content or area selected ( Supplementary Fig. 2 ). We numerically assessed the light-trapping effect of the Blu-ray structure on a typical polymer solar cell with a PTB7:PC 71 BM active layer [23] (see Supplementary Fig. 3a for the device structure) by performing one-dimensional (1D) rigorous coupled-wave analysis [24] . We modelled the absorption both parallel and perpendicular to the track, as marked by the four lines on the AFM image shown in Supplementary Fig. 3b . We calculated the corresponding absorption spectra from 315 to 775 nm both under transverse-electric ( Supplementary Fig. 3c ) and transverse-magnetic ( Supplementary Fig. 3d ) polarizations in reference to the plane of the cross-section. When compared to a non-patterned solar cell, the spectra of Blu-ray-patterned devices display broadband enhancement under both polarization conditions [16] , [25] , [26] . Extremely high enhancement 113.9% can be found in the region between 700 to 800 nm for transverse-magnetic polarization, indicating the underlying importance of the light-trapping effect in the weak absorption region of the active layer. The overall broadband absorption enhancement of a Blu-ray-patterned device, 18.2%, was calculated by averaging over these simulation results, as shown in Supplementary Fig. 3e . 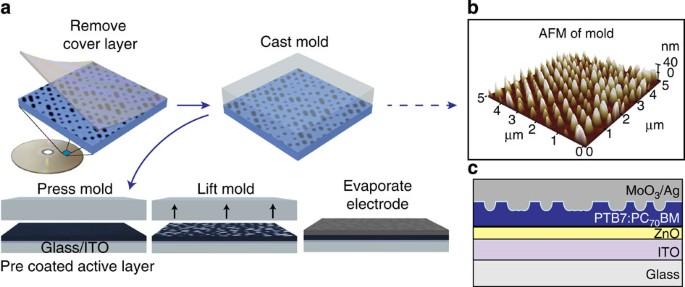Figure 2: Processing of Blu-ray-patterned solar cells. (a) Schematic diagramming the process for delaminating a BD and casting a PDMS mould on the exposed recording layer; fabricating the nanopatterned solar cells; and imprinting the active layer using the nanopatterned PDMS mould and evaporating the MoO3/Ag electrode. (b) AFM image of the nanopatterned PDMS mould. (c) Schematic diagram of the solar cell architecture used in the numerical and experimental portions of this work. Photovoltaic device fabrication and characterization Figure 2a illustrates the typical procedure for fabricating Blu-ray-patterned polymer solar cells. The BD was first delaminated to expose the pattern of pits and lands, which was replicated on a polydimethylsiloxane (PDMS) stamp. AFM image ( Fig. 2b ) of the resulting stamp confirms that it is a high-quality negative replica of the Blu-ray pattern with features as small as 150 nm across and 25 nm high. Next, the pattern was imprinted into a pre-fabricated polymer active layer by contact moulding using the stamp, followed by electrode deposition to complete the device. The final device structure is illustrated in Fig. 2c . Figure 2: Processing of Blu-ray-patterned solar cells. ( a ) Schematic diagramming the process for delaminating a BD and casting a PDMS mould on the exposed recording layer; fabricating the nanopatterned solar cells; and imprinting the active layer using the nanopatterned PDMS mould and evaporating the MoO 3 /Ag electrode. ( b ) AFM image of the nanopatterned PDMS mould. ( c ) Schematic diagram of the solar cell architecture used in the numerical and experimental portions of this work. Full size image The AFM images in Fig. 3a clearly show successful transfer of the Blu-ray pattern to the active layer after nanoimprinting, in stark contrast with a non-patterned one. Line scans ( Fig. 3a ) show that the feature sizes are highly consistent with those of both the stamp and the original BD. The transferred pattern (~1 cm 2 ) displayed uniform iridescent reflection ( Fig. 3b ), demonstrating the reliability of this nanoimprinting process over large areas. We measured the reflection ( R ) spectra of both non-patterned and Blu-ray-patterned solar cells and plotted 1− R , that is, absorption in Fig. 3c . The absorption of the Blu-ray-imprinted cell is significantly enhanced by 21.8% over the entire absorption profile. Notably, the benefit of light trapping is most pronounced after 700 nm, reaching 49.0%, where the material absorbs weakly. Both observations are consistent with the simulation shown in Supplementary Fig. 3 . The enhanced broadband absorption of Blu-ray-patterned solar cells indeed led to improved external quantum efficiencies (EQEs) ( Fig. 3d ). The overall EQE enhancement averaged over the entire absorption profile is 30.8%, while the averaged enhancement is 85.0% for wavelengths >700 nm. As a result, the patterned cells delivered 16.9% higher short-circuit current densities ( J sc ), eventually leading to a power conversion efficiency enhancement of 11.9% (see Supplementary Fig. 4 and Supplementary Table 1 for detailed performance results). Although higher J sc values have been reported for PTB7:PC 71 BM solar cells with thicker active layers (~100 nm) [23] , in the current study, an active layer thickness of 50 nm was chosen to best demonstrate the light-trapping effect while avoiding shorting caused by imprinting with the 25-nm-deep pattern. However, the depth of the pits could be modified during the mould fabrication step (for example, via etching) to accommodate the needs of alternative thicknesses for device optimization. 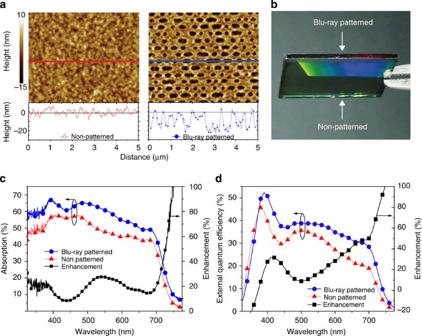Figure 3: Physical morphology and performance characteristics of Blu-ray-patterned solar cells. (a) AFM images of the active layer without stamping and after stamping with a Blu-ray-patterned mould. The horizontal line profiles illustrate the depth contrast of the Blu-ray-patterned active layer. (b) Optical images of a half-patterned solar cell showing iridescent scattering due to the periodic nature of the Blu-ray pattern. (c) Reflected absorption (1−R) measurements from a Blu-ray-patterned solar cell. (d) Measured EQEs show a broadband enhancement and agree well with the calculated absorption spectrum in (c). Figure 3: Physical morphology and performance characteristics of Blu-ray-patterned solar cells. ( a ) AFM images of the active layer without stamping and after stamping with a Blu-ray-patterned mould. The horizontal line profiles illustrate the depth contrast of the Blu-ray-patterned active layer. ( b ) Optical images of a half-patterned solar cell showing iridescent scattering due to the periodic nature of the Blu-ray pattern. ( c ) Reflected absorption (1− R ) measurements from a Blu-ray-patterned solar cell. ( d ) Measured EQEs show a broadband enhancement and agree well with the calculated absorption spectrum in ( c ). Full size image The work here demonstrated the use of pre-written, Blu-ray movie discs as extremely low-cost nanoimprinting templates for creating photon management nanostructures in thin-film solar cells. Mode analysis ( Supplementary Fig. 5 ) suggests that the Blu-ray patterns can be broadly applied for light trapping in other types of solar cells, including those made with amorphous Si, III–V and II–VI semiconductors, and perovskite compounds. In contrast to previous attempts to make use of the periodic micro/nanostructures in blank optical storage media [27] , [28] , [29] , here we take advantage of the quasi-random patterns in information-laden discs. Thus the new insight opens up promising areas, where repurposing of a low-cost consumer product leads to much higher-end, value-added applications. Fourier transforms We computed the two-dimensional (2D) discrete Fourier transform of the images in Fig. 1 (left) and customized the colour map to improve the contrast of the Fourier transform (FT) images so as to better compare the features. Numerical calculations The absorption was calculated by rigorous coupled-wave analysis, which is one of the most commonly used techniques to solve the scattering problem in Fourier space. For the multilayered dielectric stacks, Fourier expansions of both the field and the permittivity lead to an algebraic eigenvalue system for each layer. As we are interested in quasi-randomness along one direction, a 1D simulation is implemented with periodicity 10 μm. The number of Fourier components considered is 289 and the convergence test was performed on the selection of the diffraction order to ensure the numerical accuracy. Nanopatterned mould fabrication We fabricated PDMS nanopatterned moulds using a delaminated BD as the master. We first trimmed the Blu-ray movie disc (Police Story 3: Super Cop) around the edges using scissors, and then carefully peeled off the cover layer ( Fig. 1a ) to reveal the pattern shown in Supplementary Fig. 1 . No cleaning or secondary processing of the BD was required, as the cover layer effectively protects the nanopatterned surface after manufacturing. We then cast PDMS on top of the delaminated BD and cured it overnight at 60 °C. After preparation, the PDMS mould could be lifted off the BD and reused several times. It should be noted that the cover layer, which we removed as shown in Fig. 2a , contains the same pattern as the PDMS mould and can also be used as a nanoimprinting stamp. However, we found that PDMS stamps could more reliably transfer the 2D pattern to polymer thin films due to their flexibility, ductility and favourable surface energy properties. Device fabrication Figure 2 schematically shows the device fabrication procedure. We fabricated all devices on patterned ITO-coated glass substrates (20 Ω sq −1 ) that were pre-cleaned and treated with oxygen plasma immediately before use. We employed a sol–gel synthesis for the ZnO ETL following ref. 30 . We spin-coated 0.25 M zinc acetate dihydrate and 0.25 M ethanolamine in 2-methoxyethanol through a polyvinylidene difluoride filter and annealed at 180 °C for 20 min to yield a 15-nm-thick film. We verified the 15 nm thickness of the ZnO films using spectroscopic ellipsometry (J.A. Woollam M2000U). We prepared the active material by blending PTB7 (1-material) with PC 71 BM (nano-C) at 1.0:1.5 in a solution of 97 vol% chlorobenzene (Sigma) and 3 vol% diiodooctane (Sigma) and mixed for 2 days at 65 °C. A solution concentration of 10 mg ml −1 by total weight yielded an active layer thickness of 50 nm. After spin-coating, we gently placed a PDMS stamp on top of the active layer (for stamped devices) and placed all devices under vacuum for 2 h in order to allow for evaporation of the diodooctane, and for PTB7 and PC 71 BM domains to phase segregate. It should be noted that if the stamp was removed immediately the nanopattern would fade away within a few hours, which we attribute to the residual solvent allowing the active material to reconfigure into a lower-energy (that is, flatter) morphology. After carefully removing the stamp, all devices were moved to a thermal evaporator (Angstron Covap II), where we deposited 10 nm of MoO 3 (Alfa Aesar, Puratronic, 99.9995%) and 100 nm of Ag. We also conducted control experiments with devices stamped with a flat PDMS mould. The physical morphologies of the flat-stamped control and non-stamped active layers are comparable ( Supplementary Fig. 6 ), with the flat-stamped device being slightly smoother. Characterization of photovoltaic cells We performed microscopic and morphological characterization using a scanning electron microscope (FEI Nova 600) and AFM (Park Systems XE-100), respectively. We obtained reflection data with an Andor SR-303i_A spectrometer combined with Leica DMI 3000 M microscope (10 × objective, numerical aperture=0.3, 100 W halogen light source). We measured current density–voltage characteristics of all devices under AM1.5 G illumination using an Oriel Xe solar simulator, employing filters to cut off grating overtones. Correct current density measurements were calculated after measuring EQE under short-circuit conditions (Enli Technology QE-R3018). A calibrated monosilicon diode with known spectral response served as a reference. We averaged over the best 12 devices measured to obtain our device statistics. How to cite this article: Smith, A. J. et al . Repurposing Blu-ray movie discs as quasi-random nanoimprinting templates for photon management. Nat. Commun. 5:5517 doi: 10.1038/ncomms6517 (2014).